Conformational activation of talin by RIAM triggers integrin-mediated cell adhesion The membrane localization and activation of cytoskeletal protein talin are key steps to initiate the integrin transmembrane receptors’ activation, which mediates many cellular adhesive responses such as cell migration, spreading and proliferation. RIAM, a membrane anchor and small GTPase RAP1 effector, is known to bind to the C-terminal rod domain of talin (talin-R) and promote localizations of talin to the membrane. Through systematic mapping analysis, we find that RIAM also binds to the N-terminal head of talin (talin-H), a crucial domain involved in binding and activating integrins. We show that the RIAM binding to talin-H sterically occludes the binding of a talin-R domain that otherwise masks the integrin-binding site on talin-H. We further provide functional evidence that such RIAM-mediated steric unmasking of talin triggers integrin activation. Our findings thus uncover a novel role for RIAM in conformational regulation of talin during integrin activation and cell adhesion. Almost every life process involves the adhesion of cells to their surroundings, the extracellular matrix (ECM). A major mediator of such an adhesion is integrin, a heterodimeric (α/β) transmembrane receptor that binds to the ECM proteins via its large ectodomains and connect to intracellular cytoskeleton via its small cytoplasmic tails (CTs) [1] , [2] , [3] . The ability of the integrin binding to the ECM proteins is controlled by a distinct ‘inside-out’ signalling mechanism (integrin activation), that is, an agonist-induced intracellular signal induces a conformational change of integrin cytoplasmic face, which is relayed via the transmembrane region to the ectodomain, converting it from low to high-affinity ligand-binding state [1] , [2] , [3] . As a vital step for controlling all cell adhesive processes, this integrin activation process has been the subject of intensive studies for decades. A major breakthrough from these studies was the discovery of talin as an intracellular activator of integrins (for review, see refs 4 , 5 ). Talin is a large protein that can be divided into an amino-terminal (N-terminal) head (1–433, talin-H, 50 kDa) that contains a FERM domain (including F1, F2 and F3 subdomains) and a preceding F0 domain, and a carboxyl-terminal (C-terminal) rod (482–2541, talin-R, 220 kDa) that is made up of 13 consecutive helical bundles followed by a C-terminal actin-binding motif [4] , [5] ( Fig. 1a ). Extensive structural/biochemical studies have indicated that talin-H is responsible for activating integrin by disrupting the integrin α/β cytoplasmic clasp and initiating the inside-out conformational change of the receptor [6] , [7] , [8] . The key integrin-binding site is located on talin-F3. Interestingly, talin is randomly distributed [9] and autoinhibited in unstimulated cells with this integrin-binding site being masked by talin-R via an intramolecular interaction [10] , [11] , [12] . On cellular simulation, talin rapidly localizes to the plasma membrane [9] and becomes activated to bind and activate integrin [10] , [11] , [12] . Thus, talin autoinhibition and activation allow the dynamic regulation of cell adhesion processes such as cell shape change and migration. Phosphoinositol-4,5-bisphosphate (PIP2) has been shown to act as a talin activator [10] , [13] , [14] , [15] through an electrostatic ‘pull–push’ mechanism [12] . However, the specific ablation of PIP2-producing enzyme PIPKIγ in the integrin adhesion sites only partially and temporally impaired the talin-mediated cell adhesion [16] , suggesting that there are additional pathways/factors to regulate the talin activity. One emerging pathway involves small GTPase Rap1 and its effector RIAM, which was shown to engage talin in the plasma membrane and promote the integrin activation and signalling [17] , [18] , [19] , [20] , [21] , [22] . 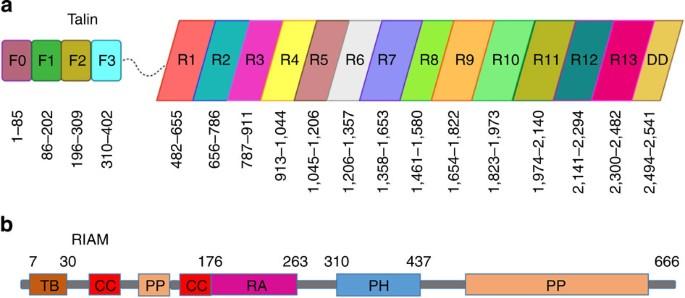Figure 1: Primary structure and domain organization of Talin and RIAM. (a) Talin: N-terminal talin head is composed of F0, F1, F2 and F3 subdomains whereas C-terminal talin-R is composed of 13 helical bundles (R1-R13) followed by a dimerization domain (DD). (b) RIAM, which comprises talin-binding site (TB), RA, PH, proline-rich domain (PP) and coiled-coil domain (CC). Figure 1: Primary structure and domain organization of Talin and RIAM. ( a ) Talin: N-terminal talin head is composed of F0, F1, F2 and F3 subdomains whereas C-terminal talin-R is composed of 13 helical bundles (R1-R13) followed by a dimerization domain (DD). ( b ) RIAM, which comprises talin-binding site (TB), RA, PH, proline-rich domain (PP) and coiled-coil domain (CC). Full size image RIAM contains a Ras association (RA) domain, a pleckstrin homology (PH) domain and a proline-rich region [17] ( Fig. 1b ). RIAM RA binds to RAP1 that attaches to the membrane and RIAM PH domain also preferentially binds to PIP2 in vivo [23] . With this combined membrane-anchoring capacity, the RAP1/RIAM complex was shown to localize talin to the plasma membrane [19] , [20] . A specific N-terminal fragment (residue 7–30, referred to as RIAM-N hereafter) of RIAM was recently found to bind to talin [20] , which plays a key role in the talin/RIAM interaction. Deletion and NMR studies have identified some RIAM-N-binding sites in talin-R in a manner analogous to vinculin binding to multiple sites of talin-R [24] . More recent crystallographic and biochemical analyses revealed two major RIAM-binding sites in talin-R, which clearly promote the talin recruitment [25] . However, the molecular basis as to how the RIAM/talin interaction ultimately triggers the integrin activation remains obscure. In this study, we undertake a detailed mechanistic investigation of the talin–RIAM interaction. Through a systematic mapping analysis, we find surprisingly that RIAM not only binds to talin-R but also to a distinct site in talin-F3. We further discover that RIAM binding to this talin-F3 site sterically occludes inhibitory talin-R, thereby freeing up talin-F3 for binding to integrin. Combined with the functional data, our findings unravel a dual role of RIAM in recruiting as well as unmasking talin for spatiotemporal regulation of integrin activation and cell adhesion. A novel RIAM-binding site on talin-F3 The talin-binding site on RIAM was previously mapped to the 1–306 containing RA domain (RIAM-1–306) and further narrowed down to the N-terminal Leu-rich region 7–30 (RIAM-N) [20] . As mentioned above, RIAM-N was recently shown to recognize multiple sites in talin-R, suggesting that multiple RIAM molecules bind to a single talin [24] , [25] with primary sites located in talin-R3 and talin-R8, respectively [25] . Consistently, we also observed that RIAM-1–306 binds to multiple fragments of talin-R (data not shown). Surprisingly, when we expanded our analysis to include talin-H, we found that, while RIAM-1–306 had no interaction with talin-F0F1 ( Fig. 2a ), it specifically bound to talin-F2F3 ( Fig. 2b ). glutathione S -transferase (GST) pull-down experiments confirmed the RIAM/talin-H interaction ( Fig. 2c ). NMR-based chemical shift mapping analysis further narrowed down the RIAM-1–306 binding to talin-F3 ( Fig. 2d ). Isothermal titration calorimetry (ITC) experiment revealed a 1:1 binding at a moderate affinity with K D ~32 μM between talin-F2F3 and RIAM-1–306 ( Fig. 2e ). Since both talin-H and full-length RIAM are membrane associated [8] , [12] , [13] once being activated, we anticipate the K D between talin-H and intact RIAM to be much stronger in the presence of cell membrane. A similar case was recently shown for the interaction between talin-H and integrin β3 CT with K D being ~438 μM in the absence of membrane [26] but becoming ~0.86 μM in the presence of membrane that binds to both talin-H and β3 CT [27] . 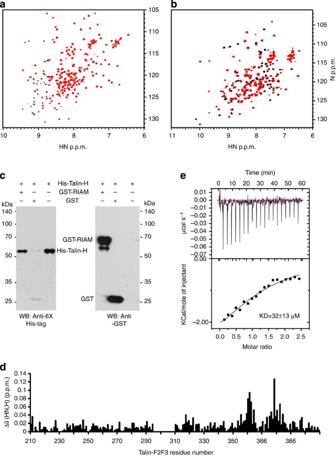Figure 2: RIAM interaction with talin-F3. (a) 2D1H-15N HSQC spectra of 40 μM15N-talin-F0F1 in the absence (black) and presence of 80 μM RIAM-1–306 (red). (b) 2D1H-15N HSQC spectra of 40 μM15N/2H-talin-F2F3 in the absence (black) and presence of 80 μM RIAM-1–306 (red). (c) Pull-down assay to show that GST-RIAM-1–306, but not GST control, binds to talin-H. (d) Chemical shift change profile of talin-F2F3 by RIAM-1–306, showing that talin-F3 is specifically perturbed by RIAM-1–306. (e)KDbetween talin-F2F3 and RIAM-1–306 by ITC. Figure 2: RIAM interaction with talin-F3. ( a ) 2D 1 H- 15 N HSQC spectra of 40 μM 15 N-talin-F0F1 in the absence (black) and presence of 80 μM RIAM-1–306 (red). ( b ) 2D 1 H- 15 N HSQC spectra of 40 μM 15 N/ 2 H-talin-F2F3 in the absence (black) and presence of 80 μM RIAM-1–306 (red). ( c ) Pull-down assay to show that GST-RIAM-1–306, but not GST control, binds to talin-H. ( d ) Chemical shift change profile of talin-F2F3 by RIAM-1–306, showing that talin-F3 is specifically perturbed by RIAM-1–306. ( e ) K D between talin-F2F3 and RIAM-1–306 by ITC. Full size image RIAM binding to talin-F3 occludes talin-R in latent talin Since previous studies have indicated that RIAM-N is the primary binding segment of talin [20] , we further examined the RIAM-N binding to talin-F2F3 as compared with RIAM-1–306. Talin-F2F3 underwent smaller chemical shift changes but with the same spectral perturbation pattern by RIAM-N as that by RIAM-1–306 ( Supplementary Fig. 1 ), suggesting that RIAM-N plays a predominant role in the RIAM/talin-F3 interaction. To understand the molecular nature of this interaction, we decided to pursue the total solution structure of talin-F3/RIAM-N complex using multidimensional heteronuclear NMR spectroscopy. With high-quality intermolecular NOEs between talin-F3 and RIAM-N ( Supplementary Fig. 2a ), we determined the talin-F3/RIAM-N interface. 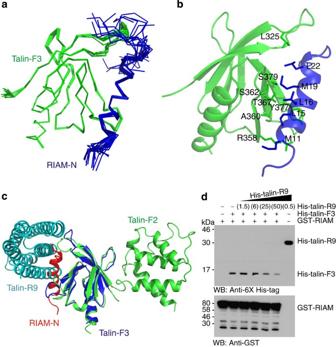Figure 3: Structure of RIAM-N/talin-F3 complex reveals a mechanism for talin unmasking. (a) Superposition of 20 calculated RIAM-N/talin-F3 complex structures with lowest energies, showing a well-defined structure. (b) Cartoon representation of the structure with the lowest energy. The side chains of the residues involved in the intermolecular interaction are displayed to demonstrate the hydrophobic interface. (c) The structure of talin-F3 (blue) bound to RIAM-N (red) was superimposed onto the talin-F2F3 (green) bound to talin-R9 (cyan), showing that RIAM-N sterically interferes with the autoinhibitory interface. (d) Pull-down assay to show that RIAM-1–306 competes with talin-R9 for binding to talin-F3. With increasing amounts (μg) of talin-R9, the population of RIAM-bound talin-F3 is reduced as visualized by the western blot analysis with anti-His (top panel). Western blot analysis of the bound GST-RIAM-1–306 with anti-GST is used as a control (bottom panel). Figure 3a shows the superposition of the 20 lowest energy structures of the talin-F3/RIAM-N complex (see structural statistics in Table 1 ). RIAM-N Q10-T23 adopts a helical conformation ( Fig. 3a and Supplementary Fig. 2b ) while the rest of the peptide is unstructured. In the complex, M11, L15, L16, M19 and L22 of the RIAM-N helix forms a hydrophobic interface with talin-F3 L325, A360, T367 methyl, methylenes of R358, S362, and S379 and side-chain of Y377 ( Fig. 3b ). Superposition of the complex structure with the crystal structure of the autoinhibited talin-F2F3/talin-R9 complex [12] shows clearly that RIAM-N would sterically interfere with the autoinhibitory interface of talin ( Fig. 3c ). This is supported by a pull-down experiment in which RIAM competes with talin-R9 for binding to talin-F3 ( Fig. 3d ). These data thus indicate that the RIAM binding to talin-F3 competes with the autoinhibitory talin-R9 for binding to talin-F3 and thereby promotes unmasking of talin to allow its binding to integrin. Figure 3: Structure of RIAM-N/talin-F3 complex reveals a mechanism for talin unmasking. ( a ) Superposition of 20 calculated RIAM-N/talin-F3 complex structures with lowest energies, showing a well-defined structure. ( b ) Cartoon representation of the structure with the lowest energy. The side chains of the residues involved in the intermolecular interaction are displayed to demonstrate the hydrophobic interface. ( c ) The structure of talin-F3 (blue) bound to RIAM-N (red) was superimposed onto the talin-F2F3 (green) bound to talin-R9 (cyan), showing that RIAM-N sterically interferes with the autoinhibitory interface. ( d ) Pull-down assay to show that RIAM-1–306 competes with talin-R9 for binding to talin-F3. With increasing amounts (μg) of talin-R9, the population of RIAM-bound talin-F3 is reduced as visualized by the western blot analysis with anti-His (top panel). Western blot analysis of the bound GST-RIAM-1–306 with anti-GST is used as a control (bottom panel). Full size image Table 1 Structural statistics of the talin-F3/RIAM-N complex. Full size table RIAM binds next to integrin site in talin-F3 to unmask talin To further understand how RIAM-N is positioned relative to integrin β CT when bound to talin-F3, we superimposed the talin-F3/RIAM-N structure with the high-resolution crystal structure of talin-F2F3/integrin β1D CT complex (PDB code 3G9W). Interestingly, Fig. 4a shows that RIAM binds to a neighbouring region of the integrin β1D CT on talin-F3, suggesting that RIAM sterically occludes talin-R9 and promotes the β CT binding to talin-F3. To experimentally investigate the ternary complex formation, we titrated excess unlabelled β3 CT into selectively 15 N-labelled RIAM-N bound to unlabelled talin-F3. 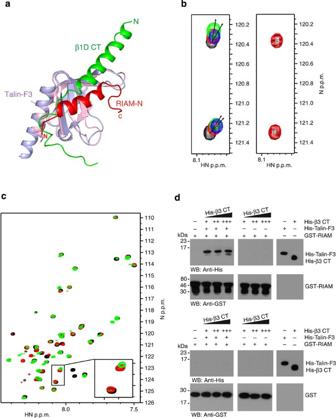Figure 4: RIAM and integrin β CT bind to neighbouring regions of talin-F3, resulting in a ternary complex. (a) Structural alignment of RIAM-N/talin-F3 complex with β1D CT/talin-F2F3 complex (PDB code 3G9W) indicates that RIAM-N (red cartoon) binds to a neighbouring region of the β1D integrin CT (green cartoon); (b) Left, HSQC overlay of 0.05 mM15N-F12,L22-RIAM-N in the absence (black) and presence of 0.2 mM talin-F3 (blue) and excess (0.4 mM in red and 1.2 mM in green, respectively) of β3 CT. The arrows indicate that on adding β3 CT, the RIAM-N resonance moves to a different direction instead of shifting back to the free-form position, suggesting the formation of a ternary complex. Right, the control HSQC spectra of 0.05 mM15N-F12,L22-RIAM peptide in the absence (black) and presence of 0.4 mM β3 CT showing that RIAM does not bind to integrin β3 CT. (c) HSQC overlay of 0.025 mM15N-labelled β3 CT in the absence (black) and presence of 0.025 mM talin-F3 (red) and 0.025 mM talin-F3 plus 0.05 mM RIAM-1–306 (green). The inset shows further line broadening or peak shifting of β3 CT resonance, which is consistent with formation of the larger ternary complex. (d) Pull-down assay to show the formation of RIAM/talin-F3/integrin β3 CT ternary complex (top left). Top middle panel shows the control that integrin β3 CT has little binding to RIAM (see alsob). GST as a control does not bind to integrin β3 CT/talin-F3 complex (lower left) and integrin β3 CT (lower middle), respectively. Figure 4b (left panel) shows that talin-F3 induced spectral changes in RIAM-N, whereas the addition of β3 CT induced still further spectral changes, demonstrating the formation of RIAM-N/talin-F3/β3 CT ternary complex (the NMR signals would shift back to free-form RIAM-N if β3 CT were to compete with RIAM-N for binding to talin-F3). As a control, we show that β3 CT has no interaction with RIAM-N (right panel in Fig. 4b ). To further verify the ternary complex formation, we examined the effect of a larger fragment of RIAM (1–306) on the mixture of 15 N-labelled β3 CT and unlabelled talin-F3. Figure 4c reveals either line broadening or peak shifting of a number of β3 CT signals, indicating the larger-sized tertiary complex formation. Consistently, our pull-down experiments showed that GST-RIAM (1–306) not only pulled down talin-F3 but also β3 CT bound to talin-F3 ( Fig. 4d ). Together these results demonstrate that RIAM-N binds to talin-F3 at the distinct site to unmask talin and promote the integrin binding to a nearby site. Figure 4: RIAM and integrin β CT bind to neighbouring regions of talin-F3, resulting in a ternary complex. ( a ) Structural alignment of RIAM-N/talin-F3 complex with β1D CT/talin-F2F3 complex (PDB code 3G9W) indicates that RIAM-N (red cartoon) binds to a neighbouring region of the β1D integrin CT (green cartoon); ( b ) Left, HSQC overlay of 0.05 mM 15 N-F12,L22-RIAM-N in the absence (black) and presence of 0.2 mM talin-F3 (blue) and excess (0.4 mM in red and 1.2 mM in green, respectively) of β3 CT. The arrows indicate that on adding β3 CT, the RIAM-N resonance moves to a different direction instead of shifting back to the free-form position, suggesting the formation of a ternary complex. Right, the control HSQC spectra of 0.05 mM 15 N-F12,L22-RIAM peptide in the absence (black) and presence of 0.4 mM β3 CT showing that RIAM does not bind to integrin β3 CT. ( c ) HSQC overlay of 0.025 mM 15 N-labelled β3 CT in the absence (black) and presence of 0.025 mM talin-F3 (red) and 0.025 mM talin-F3 plus 0.05 mM RIAM-1–306 (green). The inset shows further line broadening or peak shifting of β3 CT resonance, which is consistent with formation of the larger ternary complex. ( d ) Pull-down assay to show the formation of RIAM/talin-F3/integrin β3 CT ternary complex (top left). Top middle panel shows the control that integrin β3 CT has little binding to RIAM (see also b ). GST as a control does not bind to integrin β3 CT/talin-F3 complex (lower left) and integrin β3 CT (lower middle), respectively. Full size image Next we decided to functionally evaluate the importance of the RIAM binding to talin-F3. First, we co-expressed talin-H or full-length talin (talinFL) with RIAM, which revealed that while RIAM has no effect on the talin-H-mediated integrin activation, it substantially enhanced talinFL-mediated integrin activation, demonstrating that the talinFL activity depends on RIAM ( Fig. 5a ). Second, we made talin binding-defective RIAM mutant (M11E/F12E/L15E/L16E, RIAM-4E), which failed to induce talinFL-mediated integrin activation, further demonstrating that the RIAM binding to talinFL controls the talin activity ( Fig. 5a ). However, since the 4E mutations abolish the RIAM binding to both talin-H and talin-R, this experiment cannot distinguish the importance of RIAM binding to talin-H versus its binding to talin-R. Two possible mutagenesis approaches can be performed to address this issue: (a) point mutation in talin-H to abolish its binding to RIAM but retain the talin-R binding to RIAM; (b) point mutation in talin-R to abolish its binding to RIAM while retaining the talin-H binding to RIAM. Because the RIAM-binding site on F3 of talin-H resides in the talin autoinhibitory interface and is also very close to the integrin-binding site ( Figs 3c and 4a ), approach (a) would cause complicated effects including unmasking of talin versus reduced talin-H binding to RIAM and/or integrin. We therefore chose (b) by generating a structure-based talinFL mutant where V871 and V1540 in talin-R were both substituted into Y (talinFL-DM) to diminish the talin-R binding to RIAM [25] . 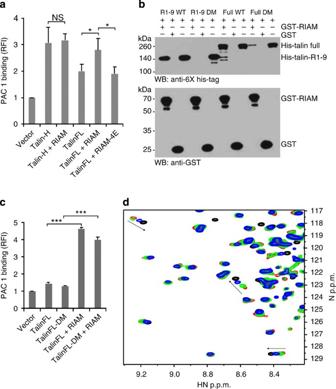Figure 5: RIAM promotes the talin unmasking and integrin activation. (a) Effects of integrin activation by talin in the presence of RIAM and talin-binding-defective RIAM M11E/F12E/L15E/L16E mutant (RIAM-4E). NS, not significant, * significant withP<0.05. The comparison clearly suggests that RIAM significantly enhanced the activation of full-length talin (talinFL+RIAM versus talinFL) but not talin-H (P>0.79, Talin-H+RIAM versus Talin-H), suggesting the role of RIAM in unmasking autoinhibited talin. The 4E mutation impairs the RIAM binding to talin and substantially reduces its activation capacity (talinFL+RIAM-4E versus talinFL+RIAM). (b) GST-based pull-down assay showing that GST-RIAM-1–306 binds to talin-R1–9 but not talin-R1–9 DM (V871Y/V1540Y) mutant. As a result, GST-RIAM-1–306 binds to talinFL but only weakly to talinFL-DM. The residual binding of talinFL-DM to RIAM may be due to talin-H/RIAM interaction as shown inFig. 1c. (c) Despite the loss of RIAM binding to talin-R, inactive talinFL-DM is still potently activated by RIAM that binds and unmasks talin-H, leading to enhanced integrin αIIbβ3 activation. *** Significant withP<0.001. The data inaandcare presented as mean±s.e.m. from three independent experiments, and the statistical significance was assessed usingt-test. (d) HSQC overlay of13C/15N-labelled 0.06 mM talin-R9 in the absence (black) and presence (red) of 0.05 mM talin-F2F3, and how this complex is dissociated by 0.5 mM 4:1 POPC:PIP2 large unilamellar vesicles (LUV) (green) as well as 0.5 mM 4:1 POPC:PIP2 LUV and 1 mM RIAM-N (blue). Considering the fact that only the outer layer of the vesicle is accessible for protein interaction, the effective concentration of PIP2 is only 0.05 mM. The arrows show that the addition of lipid alone or combination of lipid and RIAM competes with talin-R9 binding to talin-F2F3, and thus makes talin-R9 resonances move towards the free form. The combination of the lipid and RIAM is clearly more potent than the lipid alone. Figure 5b confirms that while purified talin-R1–9, which contains the major RIAM-binding sites [25] , binds to RIAM-1–306, the V871Y/V1540Y double mutations abolished the binding. As a result, purified talinFL-DM binds to RIAM-1–306 much more weakly than to wild-type (WT) talinFL ( Fig. 5b ). Remarkably, while talinFL-DM is equally inactive as WT talinFL, which is consistent with the inactive talin structure where both V871 and V1540 are outside the talin autoinhibitory domain talin-R9 (ref. 12 ), the co-expression of talinFL-DM with RIAM still potently induced the integrin activation as the co-expression of WT talinFL with RIAM ( Fig. 5c ). These data strongly indicate that while the RIAM/talin-R interaction promotes the talin recruitment to membrane, it is the RIAM/talin-H interaction that ultimately leads to integrin activation by unmasking talin. Figure 5: RIAM promotes the talin unmasking and integrin activation. ( a ) Effects of integrin activation by talin in the presence of RIAM and talin-binding-defective RIAM M11E/F12E/L15E/L16E mutant (RIAM-4E). NS, not significant, * significant with P <0.05. The comparison clearly suggests that RIAM significantly enhanced the activation of full-length talin (talinFL+RIAM versus talinFL) but not talin-H ( P >0.79, Talin-H+RIAM versus Talin-H), suggesting the role of RIAM in unmasking autoinhibited talin. The 4E mutation impairs the RIAM binding to talin and substantially reduces its activation capacity (talinFL+RIAM-4E versus talinFL+RIAM). ( b ) GST-based pull-down assay showing that GST-RIAM-1–306 binds to talin-R1–9 but not talin-R1–9 DM (V871Y/V1540Y) mutant. As a result, GST-RIAM-1–306 binds to talinFL but only weakly to talinFL-DM. The residual binding of talinFL-DM to RIAM may be due to talin-H/RIAM interaction as shown in Fig. 1c . ( c ) Despite the loss of RIAM binding to talin-R, inactive talinFL-DM is still potently activated by RIAM that binds and unmasks talin-H, leading to enhanced integrin αIIbβ3 activation. *** Significant with P <0.001. The data in a and c are presented as mean±s.e.m. from three independent experiments, and the statistical significance was assessed using t -test. ( d ) HSQC overlay of 13 C/ 15 N-labelled 0.06 mM talin-R9 in the absence (black) and presence (red) of 0.05 mM talin-F2F3, and how this complex is dissociated by 0.5 mM 4:1 POPC:PIP2 large unilamellar vesicles (LUV) (green) as well as 0.5 mM 4:1 POPC:PIP2 LUV and 1 mM RIAM-N (blue). Considering the fact that only the outer layer of the vesicle is accessible for protein interaction, the effective concentration of PIP2 is only 0.05 mM. The arrows show that the addition of lipid alone or combination of lipid and RIAM competes with talin-R9 binding to talin-F2F3, and thus makes talin-R9 resonances move towards the free form. The combination of the lipid and RIAM is clearly more potent than the lipid alone. Full size image RIAM and PIP2 orchestrate unmasking of talin Because RIAM contains a PH domain that preferentially binds to PIP2 in vivo [23] and PIP2 is a well-known promoter of talin activation [10] , [12] , [13] , we wondered if RIAM and PIP2 might act cooperatively to regulate the talin activation. This is structurally feasible since different regions of talin-H interact with RIAM and PIP2 with the former unmasking talin via steric occlusion ( Fig. 3c ) and the latter unmasking talin via the electrostatic ‘pull–push’ mechanism [12] . To experimentally examine this possibility, we performed a NMR-based competition experiment. Figure 5d shows that while PIP2-containing membrane vesicle triggers talin unmasking as shown previously [12] , the addition of RIAM-N significantly enhanced this effect, providing evidence that RIAM and PIP2 are capable of cooperating to orchestrate the potent talin activation. In this study, we have uncovered a novel regulatory mechanism of talin by RIAM. Specifically, we have shown that RIAM binds to a previously unrecognized site in talin-F3 near that for integrin binding. Using a combination of structural, biochemical and functional approaches, we further showed that the RIAM/talin-F3 interaction promotes the conformational opening of latent talin, leading to the binding and activation of integrin. By binding to the membrane-associated RAP1 via the RA domain and PIP2 via the PH domain, RIAM was previously suggested to promote the membrane co-localization of talin [19] , [20] , [23] , [25] . However, our results now suggest that RIAM has an additional key role in conformationally activating talin. The multiple binding sites of RIAM on talin-R may allow a strengthened RIAM binding to talin, thus leading to effective RIAM/talin co-localization to the membrane ( Fig. 6 ). However, it is the RIAM-N interaction with talin-H that sterically repels talin-R and leads to the talin activation ( Fig. 6 ). Such steric occlusion mechanism is distinctly different from the previously described ‘pull–push’ activation mechanism of talin by PIP2 (ref. 12 ). The presence of this RIAM pathway also explains why the ablation of the PIP2 pathway by deleting PIPKIγ at the integrin adhesion sites only partially impaired the talin-mediated cell adhesion. On the other hand, since RIAM binds to PIP2 in vivo [23] , it is possible that the RIAM and PIP2 pathways may converge at the membrane surface in certain cellular conditions to orchestrate the potent talin activation ( Fig. 6 ). Our data in Fig. 5d support this possibility. 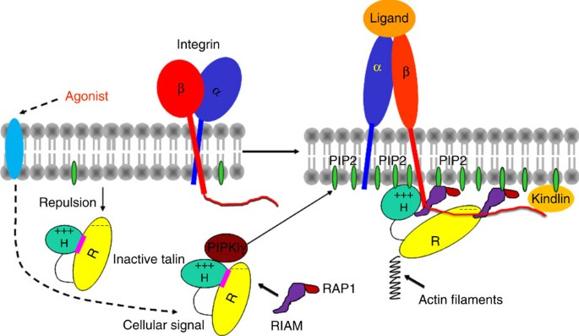Figure 6: A model of talin membrane localization and activation as mediated by the RIAM- and PIP2-mediated pathways. Upon agonist stimulation, talin is recruited to the plasma membrane by binding to localized PIP2 and/or RAP1/RIAM complex. The PIP2 binding further promotes conformational unmasking of talin via a pull-push mechanism whereas the RIAM binding promotes the talin unmasking via a steric occlusion mechanism. The two mechanisms may independently or synergistically unmask talin and regulate integrin activation. Figure 6: A model of talin membrane localization and activation as mediated by the RIAM- and PIP2-mediated pathways. Upon agonist stimulation, talin is recruited to the plasma membrane by binding to localized PIP2 and/or RAP1/RIAM complex. The PIP2 binding further promotes conformational unmasking of talin via a pull-push mechanism whereas the RIAM binding promotes the talin unmasking via a steric occlusion mechanism. The two mechanisms may independently or synergistically unmask talin and regulate integrin activation. Full size image How is the RIAM/talin interaction regulated after the integrin activation? As mentioned above, RIAM was found to bind to the overlapping sites in talin-R as vinculin—a major focal adhesion adaptor. Structural and functional analyses revealed that vinculin can displace RIAM as a switch for promoting the maturation of focal adhesions and its turnover [24] , [28] . Thus, after integrin activation, RIAM may be dissociated from talin by vinculin, triggering the focal adhesion reassembly. RIAM was also shown to regulate the subcellular localization of PLC-gamma1 that dephosphorylates PIP2 to PIP [29] , which would in turn weaken/dissociate the membrane association with talin and RIAM, respectively. Since RIAM also binds to VASP [21] —a major regulator for actin assembly, RIAM may be involved in a more complex network of cytoskeleton remodelling including talin, vinculin and VASP, which all bind to F-actin. More detailed investigation is necessary to elucidate how RIAM is spatiotemporally regulated to mediate dynamic integrin signalling and its linkage to cytoskeleton. In conclusion, we have obtained important insights into the RIAM function in regulating the integrin-mediated cell adhesion. We showed that RIAM can induce conformational opening/activation of talin, which may be also coupled with the well-known PIP2-mediated pathway for the talin activation. The finding not only defines a novel mechanism of talin activation by RIAM but also highlights how talin is under the dynamic control of a multi-faceted regulatory system to allow complex integrin signalling events, actin cytoskeleton reorganization, cell spreading and migration. Peptide and protein preparation and purification Unlabelled or 15 N-F12,L22 double-labelled peptide corresponding to residues 7–30 of RIAM was synthesized and purified by our Biotechnology Core. The longer N-terminal domain of RIAM (residues 1–306) was subcloned into the pGEX4T1 vector (GE Healthcare, Piscataway, NJ) containing a N-terminal GST tag. The protein was expressed in E. coli and purified by glutathione-Sepharose 4B resin (GE Healthcare) according to the manufacturer’s protocol. Various talin fragments including talin-F0F1 (1–205), talin-F3 (309–405), talin-F2F3 (206–405), talin-R9 (1654–1848) and remaining talin-R fragments were subcloned into pET30a vector (EMD Millipore, Danvers, MA) with a N-terminal His tag. The proteins were expressed in E. coli and purified on nickel column. After dialysing the eluted protein, the His tags were cleaved using thrombin, and the proteins were then further purified by size-exclusion chromatography [10] . A more soluble integrin β3 CT (716–762) bearing a double-mutation L 717 K/L 718 K was subcloned into pET15b vector (EMD Millipore, Danvers, MA) with a N-terminal His tag. The peptide was largely expressed in the inclusion bodies, and hence was purified under the manufacturer’s denaturation protocol followed by high-performance liquid chromatography [6] . 15 N and/or 13 C isotope labelling was achieved by employing 15 NH 4 Cl (1.1 g l −1 ) and/or 13 C glucose (3 g l −1 ) as the sole nitrogen and carbon sources in the cultures. 2 H isotope labelling was achieved by using 2 H glucose (3 g l −1 ) and preparing the culture in 99.8% D 2 O. Lipid vesicle preparation POPC (1-palmitoyl-2-oleoyl-sn-glycero-3-phosphocholine) and PIP2 were purchased from Avanti Polar Lipids (Alabaster, AL). Large unilamellar vesicles of either single or mixed lipid were prepared by extrusion. In brief, lipids were first dissolved together in chloroform. The chloroform was then removed under a stream of nitrogen followed by overnight vacuum pumping. The lipid film was hydrated in desired buffer followed by homogenization with a few freeze–thaw cycles. The Large unilamellar vesicle was finally formed by extruding the lipid suspension ~20 times through two stacked 0.1 μm polycarbonate filters (Avanti Polar Lipids). NMR spectroscopy All NMR experiments were performed at 25 °C on Bruker Avance 600 and 900 MHz spectrometers equipped with cryogenic triple resonance probes and shielded z-gradient units. Unless otherwise notified, all NMR samples were dissolved in 50 mM NaH 2 PO 4 /Na 2 HPO 4 , 50 mM NaCl, 2 mM NaN 3 , 1 mM DSS, 5% 2 H 2 O (v/v) and pH 6.8. The weighted chemical shift changes of amide proton and nitrogen were calculated using the equation: Δ δ obs[HN,N] =([Δ δ HN W HN ] 2 +[Δ δ N W N ] 2 ) 1/2 , where W HN (1.0) and W N (0.154) are weighting factors based on the gyromagnetic ratios of 1 H and 15 N. 3D 15 N-NOESY experiments were conducted with 0.5 mM protein to confirm the previously assigned resonances of Talin-F2F3 (ref. 10 ). Intermolecular NOE distance restraints for structure calculations of the talin-F3 and RIAM-N complex were obtained from 3D 15 N-NOESY spectra (mixing times 200 and 400 ms, respectively) using 15 N/100% 2 H-labelled talin-F2F3 or talin-F3 bound to unlabelled RIAM-N. 2D 15 N/ 13 C-filtered TOCSY and NOESY were performed to assign the 1 H resonances of the bound RIAM-N and to obtain intrapeptide NOEs. NMR data were processed and analysed using nmrPipe [30] , PIPP [31] and Sparky [32] . Structure calculations For the complex of RIAM-N and talin-F3, we first calculated each structure of bound form separately using Xplor-NIH standard protocols [33] with NOE distance constraints, backbone dihedral restraints that were predicted by TALOS+ (ref. 34 ), and hydrogen bonds that were automatically selected during calculations by a hydrogen bond database potential of mean force enabled through the Xplor-NIH HBDB module operating in ‘free’ mode [35] . In the next round, a group of unambiguously assigned intermolecular NOEs were incorporated for the complex structure calculation. All structures satisfying the experimental restraints converged to a single cluster. In the next iterations, the ambiguity in the intermolecular restraints was gradually reduced by examining the resulting structures so that more intermolecular NOEs were assigned. Using randomly oriented starting structures, a total of 99 final structures were calculated and the 20 lowest energy structures were chosen for analysis. A total of 1,565 intrasubunit NOEs, 160 dihedral angle constraints and 28 intermolecular NOEs led to tight convergence of the complex structure (see Table 1 for structural statistics). Structure quality was evaluated using the program PROCHECK [36] and structures are visualized with PyMOL [37] . The percentage of residues in the most favoured, generally allowed and disallowed regions of Ramachandran plot for the 20 lowest energy structures were 71.6, 27.7 and 0.7%, respectively. ITC experiment ITC experiments were performed using a Microcal iTC 200 system at 25 °C. The buffer contained 50 mM NaH 2 PO 4 /Na 2 HPO 4 , 50 mM NaCl and pH 6.8. 380 μM His-talin-F2F3 in the syringe (~40 μl) was injected 20 times in 2.0 μl aliquots into the sample-cell (~200 μl) containing 30 μM GST-RIAM-1–306 or GST or buffer only. Data were analysed by fitting to a single-site binding model with Origin Software. Pull-down assay Purified GST-fused RIAM or GST (10 μg each) was immobilized on 40 μl of glutathione-Sepharose 4B resin and equilibrated in the binding buffer consisting of 10 mM Tris, pH 7.5, 50 mM NaCl, 10% glycerol (v/v), 0.1% NP-40 (v/v) and Complete EDTA-free Protease Inhibitor (Roche, Indianapolis, IN). The desired His-tagged protein(s) were added in either GST-RIAM or GST immobilized binding mixture and incubated at 4 °C for 2 h. The beads were extensively washed for three times by the binding buffer. The bound proteins were eluted in 30 μl of 20 mM reduced glutathione (Sigma, St Louis, MO) in the binding buffer and dissolved in 30 μl of 2 × SDS sample buffer. The samples were resolved by 18% SDS–polyacrylamide gel electrophoresis and transferred onto a PVDF membrane (Millipore, Billerica, MA) for western blot analysis. The bound proteins were probed with either anti-His monoclonal antibody (120 ng ml −1 , EMD Millipore, cat. No. 70796-4) or anti-GST monoclonal antibody (0.1 μg ml −1 , Calbiochem, cat. No. OB03) and developed with Pierce ECL Western Blotting Substrate (Thermo Scientific, Portsmouth, NH). The binding experiments were performed in duplicate. Plasmids and transfections The plasmids for mouse full-length talin1, talin1-DM (V871Y/V1540Y) and talin-H were subcloned into pEGFP-N1 vector (Clontech Lab, Mountain View, CA) encoding a C-terminal red-shifted variant of WT GFP [10] . Full-length RIAM fused to EGFP was a kind gift from Dr Frank Gertler at MIT and was used to subclone RIAM-1–306 and the RIAM mutant into EGFP or dsRED vector, pDsRed-Express-N1 (Clontech Lab, Mountain View, CA). RIAM was also cloned into pCGN vector with an N-terminal HA tag. Integrin activation assay The effects of full-length talin and talin-H on integrin activation were analysed using CHO cells stably expressing integrin (αIIbβ3-CHO) and an activation-specific anti-αIIbβ3 mAb (PAC1) as described previously [10] . The effects of RIAM and talin on integrin αIIbβ3 activation were tested using the assay described previously [25] , [38] . In brief, mouse GFP talin1 alone or together with dsRED RIAM was transiently transfected into CHO cells with stably expressed integrin αIIbβ3 using Lipofectamine 2000 (Invitrogen). PAC1 binding to the different transfectants (EGFP and dsRed double-positive cells) was analysed by flow cytometry after incubating the transfected cells with anti-PAC1 mAb. Integrin activation was expressed in terms of relative median fluorescence intensities by defining the basal PAC1 binding to WT αIIbβ3 cells positive for EGFP and DsRed as 1.0. In the assay of integrin activation by TalinFL-DM, CHO cells were co-transfected with GFP-TalinFL or GFP-TalinFL–DM with HA-RIAM and harvested 24 hours after transfection. GFP positive cells were gated on to detect PAC-1 binding. The relative MFI of each transfectant was obtained by normalizing to that of the GFP empty vector transfectant, where median fluorescence intensity was defined as 1.0. The data were represented by the means±SD and the unpaired t -test was performed to calculate the P value using GraphPad software. How to cite this article: Yang, J. et al. Conformational activation of talin by RIAM triggers integrin-mediated cell adhesion. Nat. Commun. 5:5880 doi: 10.1038/ncomms6880 (2014). Accession codes : NMR structure of talin-F3/RIAM-N complex has been deposited in PDB bank ( 2MWN ).